The evolution of sex roles in birds is related to adult sex ratio Sex-role reversal represents a formidable challenge for evolutionary biologists, since it is not clear which ecological, life-history or social factors facilitated conventional sex roles (female care and male-male competition for mates) to be reversed (male care and female-female competition). Classic theories suggested ecological or life-history predictors of role reversal, but most studies failed to support these hypotheses. Recent theory however predicts that sex-role reversal should be driven by male-biased adult sex ratio (ASR). Here we test this prediction for the first time using phylogenetic comparative analyses. Consistent with theory, both mating system and parental care are strongly related to ASR in shorebirds: conventional sex roles are exhibited by species with female-biased ASR, whereas sex-role reversal is associated with male-biased ASR. These results suggest that social environment has a strong influence on breeding systems and therefore revealing the causes of ASR variation in wild populations is essential for understanding sex role evolution. One of the fundamental patterns in animal social behaviour is that females tend to be the caring sex, whereas males compete for access to females [1] , [2] , [3] . Our understanding of what determines these conventional sex roles is challenged by the reversal of sex roles in a number of organisms: the males contribute more to care than females, whereas the females compete for males [1] , [2] , [4] . In sex-role reversed species, the females are often larger and more ornamented than males, whereas the males may have specific adaptations for caring for eggs and young [2] , [4] , [5] . Sex-role reversal is taxonomically widespread occurring in insects, fishes, amphibia and birds [1] , [4] . Sex-role reversal has been a formidable puzzle for evolutionary biologists ever since Darwin [6] , because it is not clear why males under some circumstances provide most (or all) parental care, and why competition for mates should be stronger among females than among males [1] , [2] , [7] , [8] . Previous hypotheses of sex-role reversal focused on specific ecological and life-history characteristics, such as temporal and spatial variation in food resources, offspring predation and breeding dispersal [1] , [9] . Empirical evaluations, however, almost uniformly rejected these hypotheses [1] , [9] , [10] , [11] . Indeed, the life histories and ecology of sex-role reversed species are so diverse that it is hard to imagine common environmental circumstances that have led to the evolution and maintenance of sex-role reversal. Species with reversed and conventional sex roles may breed side-by-side sharing much of the environment. Examples include habitats as diverse as the Arctic tundra (phalaropes Phalaropus spp. versus calidrine sandpipers Calidris spp. [12] ) and tropical swamps (African jacana Actophilornis africanus versus lesser jacana Microparra capensis [13] ). Higher potential reproductive rates of females have been shown to correlate with more intense mating competition among females in species where only males care for the offspring [8] , although this relationship does not reveal the ecological, life-history or social predictors that have facilitated the evolution of male care in the first place. Recent theoretical models put breeding-system evolution in a different perspective by showing that ASR (expressed here as the proportion of adult males in the adult population) has a major influence on mating competition, mating systems and parental behaviour [14] , [15] . These models predict that the rarer sex is under selection to provide less care; for instance, male-biased ASR should facilitate male-biased parental care (henceforth, male care) and thus reversal of conventional parental roles, whereas female-biased ASR is predicted to favour female-biased care (henceforth, female care) [14] , [15] . Evolutionary changes in mating and parental behaviour are predicted to respond to ASR because if there are substantially more males in the population than females, males have low chances of finding a new mate. Under such circumstances, the best strategy for a male may be to provide care for the offspring, rather than desert the female after copulation and face stiff competition in acquiring a new mate. Given that the male cares and the ASR is male-biased, the females can desert the brood and acquire new mates. Testing these predictions in wild populations, however, has been challenging. The predictions are difficult to test in a single species, because most species do not exhibit sufficient variation in sex roles and ASR, although one component of sex roles, female social mating system, has been shown to correlate with ASR in dunnock Prunella modularis [16] . A multi-species comparative approach is needed, in which the variation in sex roles is compared across a set of species that differs in ASRs. However, such tests have to date been limited by the lack of data on ASR, mating system and parental care from a group of organisms that exhibit both reversed and conventional sex roles. Here we provide the first evidence that ASR correlates with parental care and social mating system consistently with the theoretical predictions using shorebirds (Scolopaci and Charadrii, sandpipers, plovers and allies). Shorebirds are eminently suitable for testing theoretical predictions of breeding-system evolution, because they exhibit unusual diversity in mating system and parental care, including some of the textbook examples of sex-role reversal [1] , [2] , [11] . We carried out a comprehensive search in primary publications, reference books and online resources for data on ASR, social mating system and parental care, with special attention to species that have been reported to exhibit sex-role reversal. We tested whether ASR predicts mating systems and parental care using Phylogenetic Generalized Least Squares [17] , [18] . Although data on ASR from wild populations are difficult to obtain [19] , the information now available for shorebirds permits tests of the theoretical predictions using statistically robust sample sizes. Relationships between ASR and components of sex roles ASR is significantly associated with social mating system: sex-role reversed species like most jacanas (Jacanidae) and greater painted-snipe Rostratula benghalensis that exhibit female polygamy and female–female competition for mates typically have strongly male-biased ASR, whereas species with male polygamy such as Northern lapwing Vanellus vanellus and ruff Philomachus pugnax have female-biased ASR. The relationships between social mating system and ASR are significant when we use polygamy frequencies ( Fig. 1a ), and a robust proxy variable for mating system, polygamy scores ( Fig. 1b ). 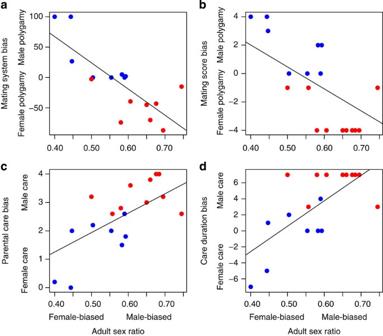Figure 1: Relationships between ASR and components of sex roles in shorebirds. ASR (number of adult males/number of adult males plus females) is associated with (a) mating system bias (% male polygamy−% female polygamy; phylogenetically correctedr=−0.79,P<0.001), (b) mating score bias (male polygamy–female polygamy;r=−0.69,P=0.001), (c) parental care bias (mean of male participation in five parental behaviour: nest building, incubation, nest guarding, chick brooding and chick guarding;r=0.70,P=0.001) and (d) care duration bias (male care duration−female care duration;r=0.69,P=0.001). Panels show species values, whereas the regression lines are fitted by PGLS models (red and blue dots represent species with reversed and conventional sex roles, respectively;n=16, 18, 18 and 18 species, respectively). Figure 1: Relationships between ASR and components of sex roles in shorebirds. ASR (number of adult males/number of adult males plus females) is associated with ( a ) mating system bias (% male polygamy−% female polygamy; phylogenetically corrected r =−0.79, P <0.001), ( b ) mating score bias (male polygamy–female polygamy; r =−0.69, P =0.001), ( c ) parental care bias (mean of male participation in five parental behaviour: nest building, incubation, nest guarding, chick brooding and chick guarding; r =0.70, P =0.001) and ( d ) care duration bias (male care duration−female care duration; r =0.69, P =0.001). Panels show species values, whereas the regression lines are fitted by PGLS models (red and blue dots represent species with reversed and conventional sex roles, respectively; n =16, 18, 18 and 18 species, respectively). Full size image Consistent with theoretical expectations, ASR also correlates with the relative contribution of sexes to parental care, because male care is associated with male-biased ASR ( Fig. 1c ). In addition, differences in the duration of care provided by males and females, another proxy for parental roles, are also significantly related to ASR ( Fig. 1d ). Sensitivity analyses These results are not sensitive to a specific phylogenetic hypothesis, or potentially confounding variables. The aforementioned results are highly consistent between alternative phylogenetic hypotheses and different branch-length assumptions: the four key tests remain highly significant by using 100 randomly selected trees from the most recent avian phylogeny [20] ( Supplementary Fig. S1 ), or using alternative phylogenies of shorebirds ( Supplementary Table S1 ). We ascertained whether the genetic mating system of shorebirds may confound the relationships between ASR, social mating system and care. However, by adding extra-pair paternity to the predictive models, the direction of relationship with ASR remains consistent in all four cases, remaining statistically significant (or marginally significant) in three out of four phylogenetically corrected correlations (mating system bias: r =−0.60, P =0.06; mating score bias: r =−0.71, P =0.02; parental care bias: r =0.66, P =0.03; care duration bias: r =0.43, P =0.11, n =10 species in all analyses). Collectively, the latter results strongly support the predicted relationships between ASR, mating system and parental care (Fisher’s combined probability test, χ 2 =24.8, d.f.=8, P =0.002). We also tested whether breeding density, the only ecological correlate of male care demonstrated previously [21] , could influence the mating system, parental care and ASR relationships. However, ASR remains strongly associated with both mating system and parental care when breeding density is added to the models ( Supplementary Table S2 ). ASR has been estimated using different methods in the field (see Methods), and we tested whether different estimation methodology may have biased the results. Nevertheless, by splitting the analyses into two subsamples (either using direct counts of breeding birds or using ASRs estimated by all other methods, see Methods) both effect sizes and the direction of relationships remain consistent with those for the whole species set. The relationships remain statistically significant (or marginally significant) in most cases ( Supplementary Table S3 ), and collectively provide a strong support for the predictions (Fisher’s combined probability test, χ 2 =46.6, d.f.=16, P <0.001). Furthermore, different detectability of the sexes, a potential confound of field estimates of ASR [19] , is not likely to bias our results: the more polygamous sex is expected to be more conspicuous because of elaborate plumage, displays and general activity [2] , which would potentially bias ASR estimates towards the direction opposite to our findings (that is, biasing ASR estimates towards the polygamous sex). Sex-specific results The relationships between mating system, parental care and ASR may be due to changes in behaviour of males, females or both sexes. We investigated these propositions by focusing on the behaviour of males and females in separate analyses. Intriguingly, the behaviour of both sexes responds to variation in ASR, because male-biased ASRs are associated with female polygamy and male care, whereas female-biased ASRs are associated with male polygamy and female care ( Fig. 2 ). 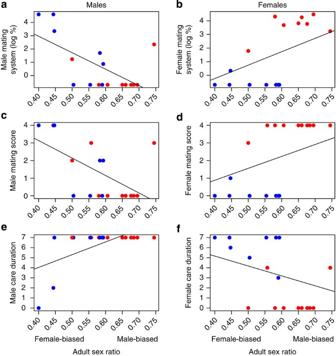Figure 2: Sex-specific relationships between ASR and sex roles. Phylogenetically corrected correlations between ASR and polygamy frequency in (a) males (r=−0.62,P=0.008) and (b) females (r=0.63,P=0.01), mating score in (c) males (r=−0.58,P=0.012) and (d) females (r=0.49,P=0.04), and care duration in (e) males (r=0.61,P=0.007) and (f) females (r=−0.50,P=0.035). Panels show species values and regression lines fitted by PGLS models (red and blue dots represent species with reversed and conventional sex roles, respectively;n=17, 16, 18, 18, 18 and 18 species, respectively). Figure 2: Sex-specific relationships between ASR and sex roles. Phylogenetically corrected correlations between ASR and polygamy frequency in ( a ) males ( r =−0.62, P =0.008) and ( b ) females ( r =0.63, P =0.01), mating score in ( c ) males ( r =−0.58, P =0.012) and ( d ) females ( r =0.49, P =0.04), and care duration in ( e ) males ( r =0.61, P =0.007) and ( f ) females ( r =−0.50, P =0.035). Panels show species values and regression lines fitted by PGLS models (red and blue dots represent species with reversed and conventional sex roles, respectively; n =17, 16, 18, 18, 18 and 18 species, respectively). Full size image Taken together, here we show for the first time that ASR is strongly associated with both social mating system and parental care across bird species, and the explanatory power of the phylogenetically corrected models is relatively high ( R 2 =0.48–0.62). Our results also reveal that both male and female behaviour show evolutionary responses to ASR, suggesting evolutionary flexibility in both mating and parental behaviour in both sexes. This is also reflected by the fact that flexible sex roles may exist even within a single species (for example, Kentish plover Charadrius alexandrinus [22] and Temminck’s stint Calidris temminckii [23] ). We propose that the evolutionary flexibility of both sexes to provide full care on their own and variation in ASR among species are among the key factors that facilitate the evolution of diverse sex roles [11] , [24] . Although in this paper we focused on sex-role reversal, our results also show that ASR is related to sex roles in general: it is associated with mating and parental behaviour through the whole range of avian sex roles, from conventional to role reversed. We conjecture that ASR may influence other aspects of social behaviour. For example, in populations with biased sex ratios homosexual pairings may be more common, and biased sex ratios may also lead to cooperative breeding where the more common sex in the population postpones dispersal, stay in the family and provide help. Further studies are needed to identify why ASR is variable across species. Biased ASRs may arise in several ways: there may be a bias in the primary sex ratio (that is, sex ratio at conception), or males and females may have differential survival during development and maturation, or as adults. Recent studies suggest that offspring sex ratio at hatching is approximately 1:1 in many birds [25] , therefore sex biases are likely to emerge after birth. It is important to emphasize that mating behaviour, parenting and sex ratios may have more dynamic relationships than currently acknowledged [15] , [26] , [27] . First, ASR can affect sex roles (see above), and conversely, reproductive behaviours can also influence mortalities and thus ASR. Following Fisher’s [28] arguments, we note that mortalities emerging from sexual competition and parental care may influence the form and intensity of these feedbacks. On the one hand, if mortality from care provisioning is high in a population with male-biased or female-biased care, this would reduce the extent of ASR bias in the population. On the other hand, if sexual selection is costly, then this may generate a positive feedback between ASR and sex roles, so that ASR may shift towards more extreme bias [15] . It is conceivable that populations can be locked in an unusual breeding system, because it is the best response to a biased ASR as generated by the breeding system itself. Intense sexual competition and care provisioning have substantial energetic and mortality costs [29] , [30] , and thus likely that ASR and sex roles can evolve quickly and concurrently in ecological time scales, rather than in a sequential manner over evolutionary time scales (for example, changes in ASR precedes changes in sex roles or vice versa ). We propose that these relationships have a complex dynamics, and the dynamics itself may contribute to the immense diversity of sex roles and breeding systems in nature. Operational sex ratio (OSR, the ratio of sexually active males to receptive females) is often used in the same context as ASR, although it has been suggested that this is mistaken [15] . OSR is only equal to ASR if the sexually active periods of adult males are identical with those of adult females. A population with male-biased ASR can exhibit female-biased OSR and vice versa . Although ASR is a demographic property of a population, OSR is also influenced by the mating and parental decisions of animals reflecting their ‘time in’ the breeding pool and ‘time out’ [8] , [15] . A significance of our present analyses is therefore to point out that a demographic property, the ratio of adult males and females, is closely correlated with mating and parenting behaviour in wild populations. ASR on its own, however, is unlikely to explain all subtle variation in mating system and parenting of animals, because these may also depend on a suite of other factors. We propose two further lines of studies to investigate the influence of ASR on sex roles. First, taxa with variable sex roles (for example, pipefish Syngnathidae, poison dart frogs Dendrobatidae and tinamous Tinamidae [4] , [5] , [8] ) are ideal groups to separate the effects of phylogenetic history, ASR, life history and ecological traits on sex-role reversal: ASR may predict sex roles in these organisms once ecology and life-history differences have been controlled for. Second, experiments are needed to manipulate ASR and investigate the corresponding changes in sex roles. Although ASR has been manipulated in the lab, experiments in natural populations, preferably in species with flexible sex roles, are required. Adult sex ratio We systematically searched for shorebirds’ ASR data in reference works (for example, birds of Western Palaearctic and birds of North America), and by extensively searching the primary literature through the Web of Knowledge (using keywords ‘shorebird*’, ‘wader*’, and English and scientific names of specific taxa such as ‘sandpiper*’ and ‘Calidris’, in combination with ‘sex ratio*’ and ‘ASR’). We calculated ASR as the ratio of adult males to all adults (males plus females) in the populations. When several estimates were available for a species, we used their mean value. In intensively studied breeding populations, ASR was often based on censuses of individually marked breeding adults. From the non-breeding period, we only included data if the ASR estimates were consistent among studies [31] , [32] , [33] . For 14 species, ASR data were taken from the original source, whereas for an additional 4 species, ASR was calculated using the data from the original sources. By restricting the analyses to the former 14 species, our results do not change qualitatively ( Supplementary Table S4 ). In two species ( Jacana spinosa and Metopidius indicus ), separate estimates were available for (i) breeding birds and (ii) breeders plus non-breeders; we repeated the analyses using both sets of data and the results remained highly consistent ( Supplementary Table S4 ). We aimed at obtaining ASR for as many shorebird species as possible, including both sex-role reversed and non-reversed species. In the main analyses ( Fig. 1a–d ), we used all ASR data (that is, mean values of all estimates regardless of the methods), whereas in the method-specific analyses ( Supplementary Table S3 ), we separated estimates into two groups (breeding censuses versus others) to maximize the number of species in the latter analysis. All data and references are provided in Supplementary Tables S5 and S6 . Social and genetic mating system We used two variables to describe social mating systems. First, we recorded the percentages of socially polygamous individuals separately for males and females [30] , using reference works and primarily literature ( Supplementary Tables S5 and S6 ). Both simultaneous and sequential polygamy were included for both sexes, and if both types of social polygamy occurred within a sex, we used their sum. If several estimates of polygamy were reported for a species, we used their mean. We considered males (or females) monogamous if social polygamy was not reported for the given sex. Lekking birds (two species P. pugnax and Scolopax minor ) do not exhibit social pair bonds, thus to express the common assumption that male–male competition is intense in lekking species [34] , we allocated 100% male polygamy for these species. We calculated mating system bias to represent the species’ social mating systems as % male polygamy−% female polygamy. We did not find data on polygamy frequency for two species ( Charadrius nivosus and Rostratula benghalensis ), so the maximal sample size for mating system bias tests is 16 species. Second, we also used mating system scores as a proxy variable of social mating systems for two reasons: (i) these scores are robust to observer errors in frequency estimates and (ii) to include the two species in the analyses (see above) that did not have frequency data available. We scored the overall incidence of polygamy for each sex on a 0–4-point scale [35] , with ‘0’ corresponding to no (or very rare) polygamy (<0.1% of individuals), ‘1’ to rare polygamy (0.1–1%), ‘2’ to uncommon polygamy (1–5%), ‘3’ to moderate polygamy (5–20%) and ‘4’ to common polygamy (> 20%). For C. nivosus and R. benghalensis , we estimated mating system scores using verbal description of their mating behaviour and pair bonds. Mating score bias was then calculated as the difference between the male and female scores. Extra-pair paternity data were collected from published sources (see Supplementary Tables S5 and S6 ) and presented as % of broods that include extra-pair offspring. Parental care We used two variables to estimate the role of the sexes in care provisioning. First, we scored the participation of males on a five-point scale (0–4) for five types of parental behaviour: nest building, incubation, nest guarding (guarding and defending the nest during incubation), chick brooding and chick guarding (guarding and defending of the brood after hatching) [30] , [35] . We did not include chick feeding because most shorebirds are precocial, so that the parents do not feed their young. We also did not include post-fledging care because many shorebirds do not care for the fledged offspring, and also because data are limited on post-fledging care. For all types of care, score ‘0’ indicated no male participation (that is, all care carried out by females), score ‘1’ indicated 1–33% male care, score ‘2’ indicated 34–66% male care, score ‘3’ indicated 67–99% male care and score ‘4’ indicated 100% male care (that is, no female care). These scores were based on quantitative data if such data were available (for example, % incubation provided by males) or on qualitative descriptions of care in the data source. For example, when a source stated that ‘most brooding is provided by females’, then brooding was scored as 1 to express the small involvement of male. We calculated parental care bias as the mean score of the five parental activities. For three species ( Actitis macularius , Coenocorypha aucklandica and Jacana jacana ) and an additional one ( R. benghalensis ), we did not find reliable data on some aspect of care, so for these species the mean score was calculated using four (or two) types of care, respectively. Our scoring expresses male care relative to female care, which is directly relevant for quantifying parental sex roles. For example, a score of 4 refers to complete parental sex-role reversal. Second, we estimated the duration of parental care for each sex according to how long the adult cared for the offspring. Following a previous comparative study [24] , the length of incubation and brood care were divided into three periods (scores 1–3 and 4–6). If a parent did not incubate, it was given a score of 0, and if it stayed until the chicks fledged, it scored 7. Sex bias in care duration was calculated as male score minus female score. In New Zealand snipe C. aucklandica both parents care, although after the hatching of the eggs the males and the females divide the brood and care for half of the brood alone. Because this is not entirely the same as biparental care of the brood exhibited by other shorebirds, we investigated the sensitivity of the results to this data point. Nevertheless, the results qualitatively remain highly consistent when this species is excluded from the analyses ( Supplementary Table S4 ). Breeding density We followed Owens [21] to obtain comparable breeding density data. We searched for maximum breeding density and took the number of nests or pairs per hectare. Then, we followed Owens’ protocol and used a 1–6-point scale [21] to convert breeding density into density scores. We used breeding density in the analyses in two ways: (i) density scores were included in multivariate models as a predictor in addition to ASR and (ii) log-transformed density was included in multivariate models together with log-transformed female body mass and ASR; body mass was included in the models because it strongly correlates with density [21] . We repeated the latter analysis with male mass and reached qualitatively consistent results with those using female mass (results not shown). Phylogenetic comparative analyses We used Phylogenetic Generalized Least Squares (PGLS) with maximum likelihood to find the best fitting λ [17] , [18] . For most analyses, we used a supertree of shorebirds [36] , from which we pruned species with missing data, and following a recent molecular phylogenetic study, we separated C. nivosus from C. alexandrinus [37] ( Supplementary Fig. S2 ). This phylogenetic hypothesis is based on recent advances in molecular phylogenetics and morphology, and has been often used in comparative studies of shorebirds. We checked the robustness of the results in two ways. First we re-run the key PGLS models using a sample of 100 trees from the most recent comprehensive avian phylogeny [20] to which we added C. nivosus as described above ( Supplementary Fig. S1 ). Second, we repeated the analyses using three alternative phylogenetic hypotheses [38] , [39] , [40] ( Supplementary Table S1 ). Because branch lengths were not available for the latter trees (either because no branch length were provided or because we added some of the species to the phylogenetic tree and hence were unable to use the original branch lengths), we used branch lengths estimated by Nee’s method as implemented in Mesquite 2.74 (refs 41 , 42 ). To assess the sensitivity of the analyses to the branch-length assumption, we repeated the analyses with unit branch length ( Supplementary Table S1 ). All analyses were carried out using the ‘caper’ package in R [43] . Correlation effect sizes were calculated from the output of the PGLS models [44] . All statistical tests were two-tailed. How to cite this article: Liker, A. et al. The evolution of sex roles in birds is related to adult sex ratio. Nat. Commun. 4:1587 doi: 10.1038/ncomms2600 (2013).